Architecture and dynamic remodelling of the septin cytoskeleton during the cell cycle Septins perform diverse functions through the formation of filaments and higher-order structures. However, the exact architecture of septin structures remains unclear. In the budding yeast Saccharomyces cerevisiae , septins form an ‘hourglass’ at the mother-bud neck before cytokinesis, which is converted into a ‘double ring’ during cytokinesis. Here, using platinum-replica electron microscopy, we find that the early hourglass consists of septin double filaments oriented along the mother-bud axis. In the late hourglass, these double filaments are connected by periodic circumferential single filaments on the membrane-proximal side and are associated with centrally located, circumferential, myosin-II thick filaments on the membrane-distal side. The double ring consists of exclusively circumferential septin filaments. Live-cell imaging studies indicate that the hourglass-to-double ring transition is accompanied by loss of septin subunits from the hourglass and reorganization of the remaining subunits into the double ring. This work provides an unparalleled view of septin structures within cells and defines their remodelling dynamics during the cell cycle. Septins are cytoskeletal proteins conserved across all animals and fungi. They were first discovered and analysed in the budding yeast, S. cerevisiae , for their function in cytokinesis [1] . Although best known for this function, septins also play important roles in cell migration, ciliogenesis, neuronal branching and other basic cellular functions, as well as in human pathologies [2] , [3] , [4] , [5] , [6] . Thus, research on septins has accelerated greatly in the past few decades, yet the ultrastructure of septin high-order assemblies in the cell remains elusive. Biochemical studies indicate that the five mitotic septins from S. cerevisiae form at least two distinct palindromic heterooctamers (Cdc11-Cdc12-Cdc3-Cdc10-Cdc10-Cdc3-Cdc12-Cdc11 and Shs1-Cdc12-Cdc3-Cdc10-Cdc10-Cdc3-Cdc12-Shs1; the third possible octamer, Cdc11-Cdc12-Cdc3-Cdc10-Cdc10-Cdc3-Cdc12-Shs1, has not been characterized in vitro ) [7] , [8] . Each octamer is estimated to be 4-5 nm in diameter and 25-32 nm in length [7] . The Cdc11-containing octamers purified from S. cerevisiae [9] or bacteria polymerize end-to-end into double filaments (or ‘paired filaments’), whereas the Shs1-containing octamers purified from bacteria form rings of single filaments [8] . Despite this wealth of in vitro work, technical challenges of imaging yeast cytoskeleton at high resolution have limited insight into septin structures in vivo . In S. cerevisiae , septins form an ‘hourglass’ at the bud neck before cytokinesis, which is then converted into a ‘double ring’ at the onset of cytokinesis [4] , [10] , [11] . Various studies have led to conflicting models of filament organization in these cellular structures. The septin hourglass was first visualized by thin-section electron microscopy (EM) as 10-nm striations perpendicular to the mother-bud axis spaced apart at regular intervals of 28 nm [12] . These striations sometimes exhibited medial gaps at high magnification. Thus, these striations were interpreted for some time to be septin double filaments encircling the bud neck. In some grazing sections, another set of filaments diagonal to the double filaments was observed. The basic observations were confirmed and further extended by a recent cryo-electron tomography study, which suggested that septin double filaments encircle the bud neck at a regular interval of ~30 nm, while single axial filaments cross-link the double filaments with irregular intervals of ~10–20 nm [13] . It is worth noting that by thin-section EM, no filaments are visible in cells undergoing cytokinesis [12] , [13] ; thus, these approaches have not been able to shed light on the structure of the double ring. In contrast to these EM studies, the septin hourglass was proposed to contain filaments ordered in parallel to the mother-bud axis, and the striations seen in thin-section EM were thought to be an artefact generated by the subunit periodicity of septin filaments [14] . Indeed, purified septins containing glutathione S -transferase-tagged Cdc11 form tight lattices of laterally associating filaments and exhibit similar striations with a periodicity of 30 nm [9] . Although this seemed like a radical idea at the time, it was later supported by the observation that cells lacking the septin regulator Gin4 displayed prominent ‘septin bars’ along the mother-bud axis [15] . This model was also corroborated by polarized fluorescence microscopy studies, which indicated that (1) filaments in the hourglass are oriented parallel to the mother-bud axis [16] , [17] and (2) filaments rotate 90° on hourglass-to-double ring conversion [16] . To determine which of the conflicting models is correct, we visualized the septin structures from unroofed spheroplasts (yeast cells with their cell wall removed while still alive) using platinum-replica EM [18] . This approach has the advantage of visualizing cytoskeletal elements in isolation from the dense cytoplasm of yeast cells, which could otherwise complicate the interpretation of electron densities into patterns of filament organization as seen in thin-section EM. It also has the advantage of visualizing cytoskeletal structures at a much higher resolution, revealing ultrastructural details (for example, filament types and organization patterns) that are otherwise missed by fluorescence light microscopy. By combining this approach with cell synchronization, genetic disruption and advanced live-cell imaging techniques, we found that the early hourglass is composed of double filaments along the mother-bud axis. Before cytokinesis, the hourglass acquires single septin filaments orthogonal to the mother-bud axis that cross-link the double filaments at a regular interval. During cytokinesis, the hourglass double filaments disassemble and reorganize into circumferential filaments to form the double-ring structure. This work settles a central debate in the septin field and establishes a new model of septin architecture and remodelling dynamics. Radial double filaments make up the early hourglass To determine the architecture of septin structures in vivo , we visualized cell cortices by platinum-replica EM [18] , [19] . In brief, these cortices were generated from unsynchronized yeast cells that were spheroplasted (cell wall removed), attached to poly-lysine-coated coverslips, unroofed and fixed. The identity of the septin structures was confirmed by correlative light and EM analysis of immunofluorescently labelled samples ( Supplementary Fig. 1a ). Out of 47 cell cortices containing septin structures, 68% of structures were composed of filaments of consistent lengths (300–400 nm) arranged parallel to one another into radial arrays (8%) or strips (60%) ( Supplementary Fig. 1b,c ), similar to the reported gauze-like structures [19] . Another 26% of structures were composed of longer filaments with variable lengths that laterally associated with one another into circular arrays (11%) or fragments (15%) ( Supplementary Fig. 1d,e ). The remaining 6% of structures had no clear organization. The ‘strips’ and ‘fragments’ are probable partial structures ( Supplementary Fig. 1c,e ) derived from the respective radial or circular arrays ( Supplementary Fig. 1b,d ) due to the change in membrane topology during spheroplasting or the orientation at which the cell was unroofed. The bias in the frequency of radial structures compared with circular structures from an asynchronous population might reflect cell cycle-dependent changes in septin organization. To examine this possibility, we analysed a population of cells synchronized to the early hourglass stage. To accomplish this, we first arrested bar1Δ cells at the unbudded stage (or at the beginning of the cell cycle) using α -factor. These cells cannot break down the α -factor and, therefore, are highly sensitive to the pheromone [20] . When nearly 100% of cells were at the unbudded stage, we washed out the pheromone, allowed the cells to enter the cell cycle and spheroplasted them once a majority reached the early hourglass stage (small to medium-budded stage). A strain carrying Cdc3-GFP was used so that synchrony could be assessed by septin localization in addition to bud morphology, although strains not expressing any fluorescent proteins were used for preparing samples for EM. Synchrony was measured after putting cells through the spheroplasting protocol without the addition of cell wall-digesting enzyme, to control for any cell cycle progression during processing, which in our experience is negligible ( Fig. 1a ). As expected, once cell wall was removed, all budded cells became spherical due to the turgor pressure ( Fig. 1b ). We achieved 72% ( n =69) synchrony at the early hourglass stage. Less than 5% of cells were in the double-ring stage, and the remaining cells were mostly unbudded with no septin hourglass. Some unbudded cells had small puncta of Cdc3-GFP in the cell cortex, which might represent remnants of the ‘septin bars’ formed in shmooing cells in response to α -factor treatment [15] . To assure that the septin bars do not account for any of the structures observed, we analysed shmooing cells with EM but did not recover a substantial number of filamentous structures. Fluorescent recovery after photobleaching (FRAP) analysis showed that the septin bars were highly dynamic ( Supplementary Movie 1 ), which might explain why these structures were not preserved during the unroofing process. This notion is further supported by the previous observation that similar dynamic ‘septin bars’ at the neck of the filamentous fungus Ashbya gossypii were not detected by thin-section transmission EM unless stabilized by forchlorfenuron [17] . 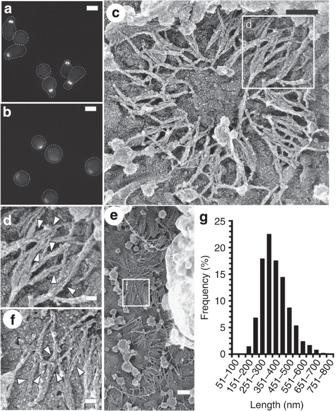Figure 1: Double filaments parallel to the mother-bud axis make up the early hourglass structure. (a,b) Fluorescence images of Cdc3-GFP inbar1Δ(YEF7170) cells identically synchronized without (a) and with (b) zymolyase treatment. Electron micrographs of cortical structures recovered from cells synchronized to the early hourglass stage (bar1Δ;YEF2497) show short double filaments organized into full (c) and partial (e) radial arrays. (d,f) Enlarged boxed regions fromcande, respectively, showing examples of double filaments (arrowheads). Scale bars, 4 μm (a,b), 200 nm (c,e) and 50 nm (d,f). (g) Distributions of individual filament lengths from early hourglass. Structures from 71 cortices were analysed. Figure 1: Double filaments parallel to the mother-bud axis make up the early hourglass structure. ( a , b ) Fluorescence images of Cdc3-GFP in bar1Δ (YEF7170) cells identically synchronized without ( a ) and with ( b ) zymolyase treatment. Electron micrographs of cortical structures recovered from cells synchronized to the early hourglass stage ( bar1Δ; YEF2497) show short double filaments organized into full ( c ) and partial ( e ) radial arrays. ( d , f ) Enlarged boxed regions from c and e , respectively, showing examples of double filaments (arrowheads). Scale bars, 4 μm ( a , b ), 200 nm ( c , e ) and 50 nm ( d , f ). ( g ) Distributions of individual filament lengths from early hourglass. Structures from 71 cortices were analysed. Full size image Remarkably, EM analysis of the synchronized cells at the early hourglass stage revealed that all identifiable structures were composed of short double filaments arranged as full ( Fig. 1c,d ) or partial ( Fig. 1e,f ) radial arrays. On occasion, long single filaments were observed laying on top of and orthogonally to the double filaments ( Supplementary Fig. 2 ). The double filaments had a thickness of 20.0±3.9 nm (mean±s.d., n =20). This measurements is consistent with previous estimates of 10 nm for double filaments [7] , given that the platinum coating and the tiny variable gap between filaments add to their thickness. Indeed, we rationalize that the platinum coat adds an additional ~8 nm to each double filament, given that the ~2-nm coat adds onto both sides of each filament in the doublet. In addition, the double filaments exhibited a narrow length distribution with a median in the 300–400 nm range ( Fig. 1g ). Such short filaments cannot encircle the bud neck (~1 μm in diameter) [21] , [22] , which is ~3,000 nm in circumference. Furthermore, their isolation as radial arrays strongly suggests that double filaments are aligned with the mother-bud axis, consistent with polarized fluorescence microscopy data [16] , [17] . Finally, the dense, parallel organization of these filaments may explain the septin immobility in the early hourglass, as revealed by FRAP analysis [23] , [24] , as well as the structural preservation through the EM protocol. Circumferential filaments make up the double ring To investigate the double-ring structure, we performed an arrest-and-release experiment to enrich cells at the correct stage of the cell cycle using the temperature-sensitive cdc15-2 mutation. Cdc15 is part of the mitotic exit network that controls the septin hourglass-to-double ring transition [11] , [25] . Thus, we first grew cdc15-2 cells at the non-permissive temperature (37 °C) to arrest them at the mitotic exit, and then released them to the permissive temperature (24 °C) to enrich cells at the double-ring stage. This procedure worked effectively, as 88% of the cells ( n =85) possessed a septin double ring, based on Cdc3-GFP localization ( Fig. 2a ). Spheroplasts generated after this treatment still contained discrete septin structures, and sometimes rings ( Fig. 2b ). Intact rings varied in radius from 500 to 900 nm ( Fig. 2c,i and Supplementary Fig. 3 ) and consisted of circumferential single and double filaments with a thickness of 9.9±2.0 ( n =13) and 20.4±3.6 nm ( n =16), respectively ( Fig. 2c–h ). Individual filaments in ring fragments varied in length but were generally longer than those in the hourglass structures, some even exceeding 3 μm ( Fig. 2j ). Thus, the double ring is composed of circumferential filaments that wrap around the bud neck, orthogonal to the mother-bud axis. Taken together, our data strongly suggest that septin filaments undergo a remarkable reorganization in length and orientation at the onset of cytokinesis. 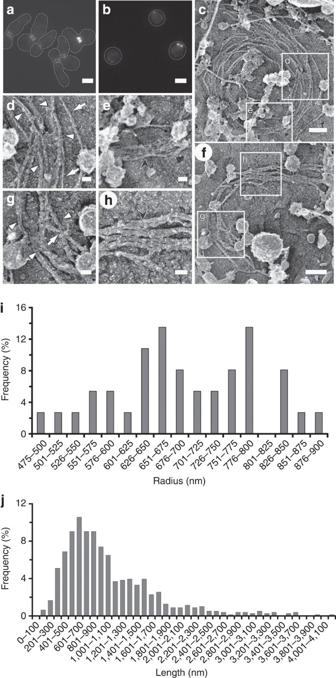Figure 2: Circumferentially arranged filaments make up the double-ring structure. (a,b) Fluorescence images of Cdc3-GFP incdc15-2(YEF7171) cells identically synchronized without (a) and with (b) zymolyase treatment. Electron micrographs of full rings (c) and ring fragments (f) among cortical structures recovered fromcdc15-2(DL3034) cells synchronized to the double-ring stage. (d,e,g,h) Enlarged boxed regions fromcandfshowing examples of single filaments (d,g, arrows), double filaments (d,g, arrowheads) and parallel arrays of multiple filaments (e,h, barbed black arrowheads). Scale bars, 4 μm (a,b), 200 nm (c,f) and 50 nm (d,e,g,h). Distributions of radii (i) (from 36 cortices) and individual filament lengths (j) (from 63 cortices) from double-ring structures. Filament dimensions were manually quantified. Figure 2: Circumferentially arranged filaments make up the double-ring structure. ( a , b ) Fluorescence images of Cdc3-GFP in cdc15-2 (YEF7171) cells identically synchronized without ( a ) and with ( b ) zymolyase treatment. Electron micrographs of full rings ( c ) and ring fragments ( f ) among cortical structures recovered from cdc15-2 (DL3034) cells synchronized to the double-ring stage. ( d , e , g , h ) Enlarged boxed regions from c and f showing examples of single filaments ( d , g , arrows), double filaments ( d , g , arrowheads) and parallel arrays of multiple filaments ( e , h , barbed black arrowheads). Scale bars, 4 μm ( a , b ), 200 nm ( c , f ) and 50 nm ( d , e , g , h ). Distributions of radii ( i ) (from 36 cortices) and individual filament lengths ( j ) (from 63 cortices) from double-ring structures. Filament dimensions were manually quantified. Full size image Radial and circumferential filaments in the transition To define the transitional forms from radial arrays to circumferential rings, we analysed populations of cdc15-2 cells arrested at mitotic exit without subsequent release. Many of the cells appeared to contain a partially split septin hourglass ( Fig. 3a ), suggestive of very slow cell cycle progression (not an absolute block) in this mutant even at the non-permissive temperature, which is consistent with a previous observation [26] . After the removal of cell wall, spheroplasts still contained discrete septin structures ( Fig. 3b ). EM analysis showed a higher proportion of disordered structures (that is, no clear organization pattern can be deduced) from these cells (27%, n =86) than cells synchronized at the early hourglass stage (0%, n =82) ( Supplementary Fig. 4 ). However, we frequently observed a novel, recurring arrangement that consisted of three kinds of filaments ( Fig. 3c–j ). First, there were strips of parallel double filaments of 300–400 nm in length (green) and 17.2±3.5 nm ( n =22) in thickness, reminiscent of those observed at the early hourglass stage. These are probably arranged along the mother-bud axis ( Fig. 3k ). Second, we found long, thick filaments (magenta) with a thickness of 34.2±6.8 nm ( n =16) that ran orthogonal to the double filaments, along points of their origin. The thick filaments were rough in outline and were located on the internal, membrane-distal side of double filaments ( Fig. 3g–i ). Third, we found a set of single filaments (orange) that also ran orthogonally to double filaments at a regular interval of 28.7±9.5 nm ( Fig. 3l ). These ‘linker’ filaments were 9.3±1.2 nm ( n =20) in thickness, similar to the single filaments in the septin double ring, and were located on the membrane-proximal side of the double filaments ( Fig. 3c,j ). The orientation ( Fig. 3c–j ) and length distributions ( Fig. 3m ) of the thick and linker filaments strongly suggest that both structures circumferentially wrap around the bud neck ( Fig. 3k ), similar to the filaments observed at the later double-ring stage. 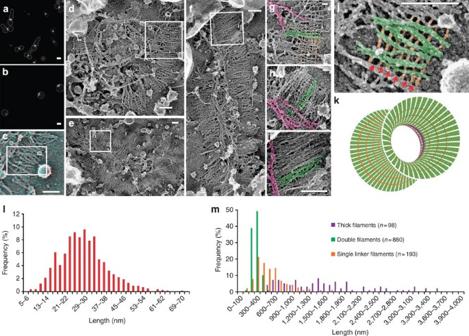Figure 3: Three sets of filaments are present during hourglass-to-double ring transition. (a,b) Fluorescence images of Cdc3-GFP incdc15-2(YEF7171) cells identically synchronized without (a) and with (b) zymolyase treatment. (c) Stereo pair images taken at ±10° are presented as an anaglyph image to show that parallel double filaments are associated with underlying single filaments. Use red-cyan anaglyph glasses with red eye at left to view 3D images. (d–f) Electron micrographs of filament-dense, organized structures fromcdc15-2(DL3034) cells arrested just before hourglass splitting. (g–i) High-magnification views of the boxed regions ind–fshowing the three classes of filaments: parallel double filaments (green), thick circumferential filaments (magenta) and single circumferential linker filaments (orange). (j) High-magnification view of the boxed region incshowing the regular spacing between single, linker filaments. (k) A model for filament arrangement in the hourglass-to-double ring transition structure, showing double filaments (green) parallel to the mother-bud axis, and thick (magenta) and single (orange) filaments wrapping around the bud neck. Thick filaments are located interiorly and centrally in the neck, while single linker filaments are most closely apposed to the cell membrane and located outside of the thick filaments. Scale bars, 4 μm (a,b), 200 nm (c–f,i,j) and 50 nm (g,h). Distributions of the distances between single linker filaments (n=906) (l) and of individual filament lengths for the three filament types (m). Dimensions of the septin structures from 22 cell cortices were manually quantified. Figure 3: Three sets of filaments are present during hourglass-to-double ring transition. ( a , b ) Fluorescence images of Cdc3-GFP in cdc15-2 (YEF7171) cells identically synchronized without ( a ) and with ( b ) zymolyase treatment. ( c ) Stereo pair images taken at ±10° are presented as an anaglyph image to show that parallel double filaments are associated with underlying single filaments. Use red-cyan anaglyph glasses with red eye at left to view 3D images. ( d – f ) Electron micrographs of filament-dense, organized structures from cdc15-2 (DL3034) cells arrested just before hourglass splitting. ( g – i ) High-magnification views of the boxed regions in d – f showing the three classes of filaments: parallel double filaments (green), thick circumferential filaments (magenta) and single circumferential linker filaments (orange). ( j ) High-magnification view of the boxed region in c showing the regular spacing between single, linker filaments. ( k ) A model for filament arrangement in the hourglass-to-double ring transition structure, showing double filaments (green) parallel to the mother-bud axis, and thick (magenta) and single (orange) filaments wrapping around the bud neck. Thick filaments are located interiorly and centrally in the neck, while single linker filaments are most closely apposed to the cell membrane and located outside of the thick filaments. Scale bars, 4 μm ( a , b ), 200 nm ( c – f , i , j ) and 50 nm ( g , h ). Distributions of the distances between single linker filaments ( n =906) ( l ) and of individual filament lengths for the three filament types ( m ). Dimensions of the septin structures from 22 cell cortices were manually quantified. Full size image In summary, the filament arrangement at the hourglass-to-double ring transitional stage suggests that double filaments, first organized along the mother-bud axis, become overlaid on their membrane-proximal side with single linker filaments and on their membrane-distal side with thick rough filaments ( Fig. 3k ). Thick filaments in the transition are Myo1-dependent The location and morphology of the thick filaments led us to speculate that they contain myosin-II. In support of this idea, FRAP analysis indicates that Myo1, the sole myosin-II heavy chain in budding yeast, is mobile at the division site before anaphase but becomes immobilized from anaphase to the end of cytokinesis [27] . This immobility depends on a putative assembly domain at the carboxy terminus of Myo1, suggesting that Myo1 might undergo cell cycle-regulated filament assembly [27] . This could also explain why our EM analysis failed to detect the thick filaments in the early hourglass (formed before anaphase). To test this possibility, we examined the transitional hourglass from synchronized myo1Δ cdc15-2 cells by EM. The mutant cells showed apparent defects in cytokinesis, as indicated by the formation of cell clusters at both permissive and non-permissive ( Fig. 4a ) temperatures. Some of the cell clusters, even when grown at the non-permissive temperature for cdc15-2 , displayed a putative transitional hourglass between two large cellular compartments, as well as a putative early hourglass between a large and a small cellular compartment ( Fig. 4a , arrow), suggesting that deletion of MYO1 causes either faster cell cycle progression or slower bud growth at 37 °C. Septin organization was also more defective in the double mutant than in the cdc15-2 cells, especially after the removal of the cell wall ( Fig. 4b ). These light microscopic observations were confirmed and extended at much higher resolution by our EM analysis. Among 92 cortices examined, 28% displayed features of a transitional hourglass (double filaments cross-linked by perpendicular single filaments) ( Fig. 4c,d ), 42% resembled the early hourglass (strips of compacted double filaments without obvious linker filaments) ( Fig. 4e,f ), 5% had both the early and the transitional hourglasses in the same cortex ( Fig. 4g,h ) and 24% were highly disordered or had too sparse of filaments to be classified. Strikingly, the thick filaments were never observed in any of the cortices examined ( Fig. 4c–k ), suggesting that their assembly completely depends on Myo1. Instead, on occasion, we observed smooth, thin and long filaments with the thickness of 10.7±1.6 nm ( n =17), which ran orthogonal to the double filaments ( Fig. 4i–k ). Similar filaments were also observed occasionally in the early hourglass ( Supplementary Fig. 2 ). The size, morphology and location of these filaments are consistent with them being actin filaments. Taken together, these data suggest that the thick filaments are made of myosin-II and, in addition, they are required for maintaining appropriate septin architecture. 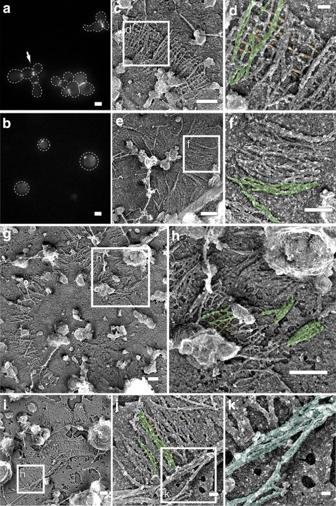Figure 4: Thick filaments are absent inmyo1Δcells arrested at the transition. (a,b) Fluorescence images of Cdc3-GFP inmyo1Δ cdc15-2(YEF7487) cells identically synchronized at the transition stage without (a) and with (b) zymolyase treatment. (c–k) Electron micrographs of structures frommyo1Δ cdc15-2(YEF7486) cells arrested at the transition stage. (c,d) A transition structure with septin double filaments (green) cross-linked with single filaments (orange), but no rough thick filaments. (e,f) An early hourglass structure with only parallel double filaments. (g) Cell cortex with both transition (left inh) and early hourglass (right inh) structures. (i) A transition structure with smooth thin filaments laying on top of and orthogonal to septin double filaments, pseudo-coloured teal at high magnification inj,k. Boxed regions inc,e,gare shown at higher magnification ind,f,h, respectively. Scale bars, 4 μm (a,b), 500 nm (g), 200 nm (c,e,f,h,i), 50 nm (d,j) and 25 nm (k). Figure 4: Thick filaments are absent in myo1Δ cells arrested at the transition. ( a , b ) Fluorescence images of Cdc3-GFP in myo1Δ cdc15-2 (YEF7487) cells identically synchronized at the transition stage without ( a ) and with ( b ) zymolyase treatment. ( c – k ) Electron micrographs of structures from myo1Δ cdc15-2 (YEF7486) cells arrested at the transition stage. ( c , d ) A transition structure with septin double filaments (green) cross-linked with single filaments (orange), but no rough thick filaments. ( e , f ) An early hourglass structure with only parallel double filaments. ( g ) Cell cortex with both transition (left in h ) and early hourglass (right in h ) structures. ( i ) A transition structure with smooth thin filaments laying on top of and orthogonal to septin double filaments, pseudo-coloured teal at high magnification in j , k . Boxed regions in c , e , g are shown at higher magnification in d , f , h , respectively. Scale bars, 4 μm ( a , b ), 500 nm ( g ), 200 nm ( c , e , f , h , i ), 50 nm ( d , j ) and 25 nm ( k ). Full size image Shs1 deletion disrupts architecture of the transition We hypothesized that the circumferential linker filaments in the transitional hourglass are made of Shs1-containing septin complexes. This is based on two lines of evidence. First, purified Cdc11-containing octamers are known to polymerize into long double filaments, while Shs1-containing octamers form rings of single filaments [8] , [9] , [28] . Second, when the two types of septin octamers are mixed in an appropriate ratio, long paired filaments are connected by electron densities at the interval of an octamer length (33±3.0 nm) [8] , which is remarkably similar to the periodicity at which the linker filaments intersect the double filaments in the transitional hourglass. To test this possibility, we examined the transitional hourglass from synchronized shs1Δ cdc15-2 cells by EM, and noted four clear features immediately. First, the overall septin organization was more defective in the double mutant than in cdc15-2 cells. However, unlike the myo1Δ cdc15-2 cells this double mutant did not display cell clusters with both transitional and early hourglasses. Septin fragments were frequently observed at the bud neck before the removal of the cell wall ( Fig. 5a ), as reported previously [8] , [29] . Septin structures were still present after spheroplasting ( Fig. 5b ). EM analysis showed that 100% of the cortices examined ( n =96) displayed disordered septin structures ( Fig. 5c–h ). Among them, 77% had highly disordered structures ( Fig. 5c,d ), that is, the basic architecture of (or the organization pattern of the three types of filaments) in the transitional hourglass was lost. The remaining 23% showed clear features of a transitional hourglass in certain regions despite overall abnormal organization ( Fig. 5g,h ). Second, myosin-II thick filaments were frequently mislocalized with respect to the septin structure. Abnormal rings and/or aggregates of thick filaments were associated asymmetrically with the disorganized septin structure ( Fig. 5e,f ), which is consistent with the previous observation that Myo1 and several other cytokinesis proteins are often mislocalized as a spot at one side of the bud neck in shs1Δ cells [30] . Third, the double filaments were often longer than in cdc15-2 cells ( Fig. 5c,d cf . Fig. 3c–j ), which corroborates with the reported presence of long septin fragments or bars at the bud neck of cells undergoing cytokinesis [29] . Finally, and most importantly, the linker filaments were observed at a much lower frequency in the double mutant than in cdc15-2 cells ( Fig. 5c–h ). Therefore, the other septin subunits can form linker filaments without Shs1 to only a small degree. Perhaps, in the absence of Shs1, Cdc11 can substitute Shs1 to form the linker filaments with limited capacity, as these septin subunits are most closely related in terms of septin complex assembly and function [8] , [30] . Together, these data suggest that Shs1 is required for efficient assembly of the linker filaments, length control of the double filaments, proper localization and/or organization of the thick filaments and, not surprisingly, the overall architecture of the transitional hourglass. 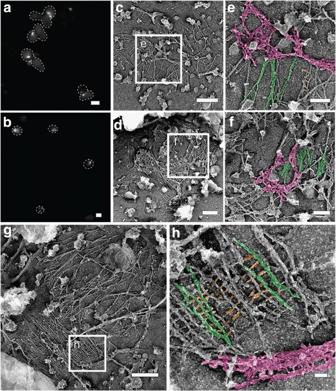Figure 5: Transition structures are disorganized inshs1Δcells. (a,b) Fluorescence images of Cdc3-GFP inshs1Δ cdc15-2(YEF7453) cells identically synchronized at the transition stage without (a) and with (b) zymolyase treatment. (c–h) Electron micrographs of structures fromshs1Δ cdc15-2(YEF7406) cells arrested at the transition stage. (c,d) Structures with disorganized myosin (magenta) and septin filaments (green). (g) Structure with general disorganization but with transition-like lattices of double (green) and single (orange) septin filaments and adjacent myosin filaments (magenta). Boxed regions inc,d,gare shown at higher magnification ine,f,h, respectively. Scale bars, 4 μm (a,b), 500 nm (c,d,g), 200 nm (e,f) and 50 nm (h). Figure 5: Transition structures are disorganized in shs1Δ cells. ( a , b ) Fluorescence images of Cdc3-GFP in shs1Δ cdc15-2 (YEF7453) cells identically synchronized at the transition stage without ( a ) and with ( b ) zymolyase treatment. ( c – h ) Electron micrographs of structures from shs1Δ cdc15-2 (YEF7406) cells arrested at the transition stage. ( c , d ) Structures with disorganized myosin (magenta) and septin filaments (green). ( g ) Structure with general disorganization but with transition-like lattices of double (green) and single (orange) septin filaments and adjacent myosin filaments (magenta). Boxed regions in c , d , g are shown at higher magnification in e , f , h , respectively. Scale bars, 4 μm ( a , b ), 500 nm ( c , d , g ), 200 nm ( e , f ) and 50 nm ( h ). Full size image The septin hourglass-to-double ring conversion To determine how the gauze-like transitional structure could generate the double ring of purely circumferential filaments, we directly assessed septin dynamics during this transition. Using Cdc3-GFP, we photobleached half of the hourglass during anaphase and visualized the fluorescence recovery until the end of cytokinesis ( Fig. 6a–g , and Supplementary Movie 2 ). Two patterns of fluorescence changes were observed. First, before the onset of cytokinesis, low levels of recovery were restricted to the ends of the hourglass, leaving a gap in the middle, resembling a double-ring arrangement ( Fig. 6b,e,g ). This data suggests that the ends of the hourglass provide spatial instruction for double-ring assembly. Indeed, the anillin-like protein Bud4 localizes to the ends of the hourglass and is required for the assembly and/or maintenance of the septin double ring, especially for the ring on the mother side [31] . Second, the signal in the unbleached half decreased rapidly in situ before the onset of cytokinesis, indicating the occurrence of filament disassembly ( Fig. 6a,b ). Indeed, ~25–50% of total septin subunits is lost from the bud neck during this transition [24] , [31] . At the onset of cytokinesis, the two halves were equal in fluorescence intensity ( Fig. 6f,g ), suggesting that septin subunits are mobile within the double ring, at least during its formation. This notion is further supported by the observation that when half of the hourglass was photoconverted, the converted (red) and unconverted (green) subunits did not intermix greatly until the onset of cytokinesis ( Supplementary Movie 3 ). The overall septin behaviours during the hourglass-to-double ring transition revealed by FRAP analysis are stereotypical for all the cells examined ( n =9) ( Fig. 6b , Supplementary Movie 2 and cell #1 presented in Fig. 6a,c–g ). Similar conclusions were reached with the photoactivation experiments ( Fig. 6h–m and Supplementary Movie 4 ). In an attempt to directly visualize the changes in filament organization during the transitional stage, we performed super-resolution three-dimensional structured illumination microscopy (3D-SIM) in live cells ( Fig. 6n , Supplementary Fig. 5 and Supplementary Movie 5 ). Cdc3-GFP appeared to be mainly organized as filamentous structures in parallel to the mother-bud axis in the hourglass ( Fig. 6n , time points 1–2) and then disassembled from the middle of the hourglass while reassembling into a double ring at the ends of the hourglass ( Fig. 6n , time points 3–9) (note that the faint ‘ring’ within the double ring and the weak ‘honeycomb’ surrounding the septin structures are typical optical artefacts associated with 3D-SIM). Taken together, these data indicate that septin hourglass-to-double ring conversion involves spatially defined filament disassembly and reassembly. This process is accompanied by a 90° change in filament orientation, which is supported by polarized fluorescence microscopy studies [16] , [17] . 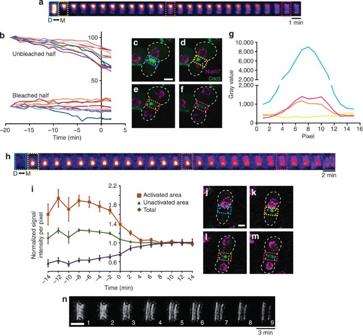Figure 6: Septin hourglass-to-double ring conversion is accompanied by filament disassembly and reassembly. (a–g) Fluorescence recovery of Cdc3-GFP (YEF6021) after its photobleaching in one half of the hourglass in cells at anaphase. (a) Frames from time-lapse sequence at 1-min intervals. M and D, mother and daughter side of the bud neck, respectively. ‘Fire’ lookup table in ImageJ was used to colour Cdc3-GFP. (b) Changes in average fluorescence intensities of Cdc3-GFP over time in the bleached and unbleached areas shown as % of pre-bleaching intensities in those areas; data on nine individual cells are shown here (seeSupplementary Movie 2). The unbleached values are normalized to 100% and the bleached values are normalized to an arbitrary 20% to avoid reaching negative values. (c–f) Whole-cell images showing the cell outline (dashed line), Cdc3 (green) and Nup57 (a component of the nuclear pore complex that marks the nuclear position, magenta) corresponding to the colour-coded time points ina: (c) pre-bleach (blue), (d) post-bleach (yellow), (e) recovery before the onset of cytokinesis (orange) and (f) recovery at or shortly after the onset of cytokinesis (pink). (g) Line-scan profiles across the bleached region inc–f. (h–m) Redistribution of Cdc3-yEPA-GFP (YEF7332-1) photoactivated in one half of the hourglass in cells at anaphase. (h) Frames from time-lapse sequence at 2-min intervals. The ‘Fire’ lookup table in ImageJ was used to colour the photoactivated Cdc3. (i) Changes in normalized pixel intensity of Cdc3-yEPA-GFP over time in activated, not activated and total bud-neck areas shown as an average of five cells. (j–m) Whole-cell images showing the cell outline (dashed line), Cdc3 (green) and Nup57 (magenta) corresponding to the colour-coded time points inh: (j) pre-activation (blue), (k) post-activation (yellow), (l) before the onset of cytokinesis (orange) and (m) at or shortly after the onset of cytokinesis (pink). (n) A representative time-lapse sequence of Cdc3-GFP (YEF6021) dynamics at 3-min intervals from anaphase through cytokinesis using 3D-SIM. Three other examples are shown inSupplementary Fig. 5. The faint honeycomb surrounding the septin structures and the ‘third ring’ in the middle are artefacts associated with this technology. Scale bars, 2 μm (c,j); 1 μm (n). Time point ‘0’ inbandirefers to the point where the two nuclei reach maximum separation. Error bars represent s.e.m. Figure 6: Septin hourglass-to-double ring conversion is accompanied by filament disassembly and reassembly. ( a – g ) Fluorescence recovery of Cdc3-GFP (YEF6021) after its photobleaching in one half of the hourglass in cells at anaphase. ( a ) Frames from time-lapse sequence at 1-min intervals. M and D, mother and daughter side of the bud neck, respectively. ‘Fire’ lookup table in ImageJ was used to colour Cdc3-GFP. ( b ) Changes in average fluorescence intensities of Cdc3-GFP over time in the bleached and unbleached areas shown as % of pre-bleaching intensities in those areas; data on nine individual cells are shown here (see Supplementary Movie 2 ). The unbleached values are normalized to 100% and the bleached values are normalized to an arbitrary 20% to avoid reaching negative values. ( c – f ) Whole-cell images showing the cell outline (dashed line), Cdc3 (green) and Nup57 (a component of the nuclear pore complex that marks the nuclear position, magenta) corresponding to the colour-coded time points in a : ( c ) pre-bleach (blue), ( d ) post-bleach (yellow), ( e ) recovery before the onset of cytokinesis (orange) and ( f ) recovery at or shortly after the onset of cytokinesis (pink). ( g ) Line-scan profiles across the bleached region in c – f . ( h – m ) Redistribution of Cdc3-yEPA-GFP (YEF7332-1) photoactivated in one half of the hourglass in cells at anaphase. ( h ) Frames from time-lapse sequence at 2-min intervals. The ‘Fire’ lookup table in ImageJ was used to colour the photoactivated Cdc3. ( i ) Changes in normalized pixel intensity of Cdc3-yEPA-GFP over time in activated, not activated and total bud-neck areas shown as an average of five cells. ( j – m ) Whole-cell images showing the cell outline (dashed line), Cdc3 (green) and Nup57 (magenta) corresponding to the colour-coded time points in h : ( j ) pre-activation (blue), ( k ) post-activation (yellow), ( l ) before the onset of cytokinesis (orange) and ( m ) at or shortly after the onset of cytokinesis (pink). ( n ) A representative time-lapse sequence of Cdc3-GFP (YEF6021) dynamics at 3-min intervals from anaphase through cytokinesis using 3D-SIM. Three other examples are shown in Supplementary Fig. 5 . The faint honeycomb surrounding the septin structures and the ‘third ring’ in the middle are artefacts associated with this technology. Scale bars, 2 μm ( c , j ); 1 μm ( n ). Time point ‘0’ in b and i refers to the point where the two nuclei reach maximum separation. Error bars represent s.e.m. Full size image A major mission of biological research is to understand the structure-function relationships in different physiological settings at different resolutions. Various high-order septin structures, including rings, spirals and other cortical structures, play important roles in diverse cellular functions including, but not limited to, cell division, spermiogenesis, neuronal spine morphogenesis, ciliogenesis, bacterial infection and cell migration [2] , [3] , [4] , [5] , [6] . However, past work on septin structures is largely at the level of description based on light fluorescence microscopy studies. Even for S. cerevisiae where pioneering work on septin structure and function has been performed, there is a central debate regarding filament arrangement in the septin hourglass and the mechanism of filament orientation change during the hourglass-to-double ring transition. Thin-section EM and EM tomography studies suggest that the paired filaments encircle the bud neck, which are intersected by orthogonal single filaments [12] , [13] . In contrast, polarized fluorescence microscopy studies suggest that the paired filaments are oriented in parallel to the mother-bud axis [16] , [17] . Furthermore, one polarized fluorescence microscopy study suggests that filaments rotate 90° during the hourglass-to-double ring transition [16] , whereas the other study suggests that the 90° change in filament orientation involves filament disassembly and reassembly [17] . Our study settles these controversial issues and, in addition, provides an unparalleled view of the septin structures in budding yeast. Collectively, our data lead us to a new model for septin architecture and dynamics during the cell cycle ( Fig. 7 ). Coincident with bud emergence or shortly after, the nascent septin hourglass consists of a radial array of double filaments organized in parallel to the mother-bud axis. In late anaphase or telophase, a more mature hourglass consists of two mirror-symmetrical arrays of double filaments connected by single filaments orthogonally at the interval of a septin-octamer length. Efficient assembly of the single filaments depends on Shs1. Myo1-dependent thick filaments are located between the septin arrays (not depicted in Fig. 7 ). At the onset of cytokinesis, the double filaments disassemble. Some subunits depart from the bud neck, while others reassemble into double filaments that join the pre-existing single filaments, guided by spatial cues from the ends of the hourglass, to form the double ring. This model can help us formulate a number of key questions regarding septin architecture, regulation and function that will be addressed in the future. 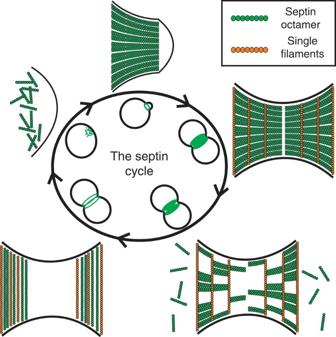Figure 7: A model of septin architecture and remodelling dynamics during the cell cycle. See text for details. Figure 7: A model of septin architecture and remodelling dynamics during the cell cycle. See text for details. Full size image In summary, our study clarifies the basic septin architecture and defines a remodelling mechanism for septin structures in budding yeast. These data will serve as a new platform on which to build a better understanding of these intricate filament organizations in various organisms. Yeast strains and culture conditions All strains used in this study are listed in Supplementary Table 1 . Cells were cultured either in rich media YM-1 (ref. 32 ) or synthetic complete (SC) minimal media lacking specific amino acid(s) [33] . New strains were made either by integrating a plasmid carrying a modified gene at a genomic locus or by transferring a deletion or tagged allele of a gene from one strain to another via PCR-amplifying and yeast transformation. Plasmid constructions All primers were purchased from Integrated DNA Technologies. Plasmid YIp211-CDC3-yEPA-GFP is the same as YIp211-CDC3-GFP [23] , except that the GFP ORF (open reading frame) was replaced by yEPA-GFP ORF encoding a photoactivatable enhanced green fluorescent protein [34] , in which the codon usage was optimized for budding yeast. Plasmid YIp211-CDC3-yEPA-GFP (integrative, URA3 ) harbours an amino-terminally yEPA-GFP-tagged CDC3 under the control of its own promoter. YIp211-CDC3-yEPA-GFP was used for yeast transformation after digestion with BglII. The plasmid is integrated at the CDC3 locus on the genome. Plasmid YIp128-CDC3-ymEos3.2 is the same as YIp128-CDC3-GFP [35] , except that the GFP ORF was replaced by the ymEos3.2 ORF encoding a monomeric photoconvertible fluorescent protein mEos3.2 (ref. 36 ), in which the codon usage was optimized for budding yeast. Plasmid YIp128-CDC3-ymEos3.2 (integrative, LEU2 ) harbours an N-terminally ymEos3.2-tagged CDC3 under the control of its own promoter. YIp128-CDC3-ymEos3.2 was used for yeast transformation after digestion with BglII. The plasmid is integrated at the CDC3 locus on the genome. Cell culture and synchronization For unsynchronized culture, wild-type (YEF473A) and CDC3-GFP (YEF5995) cells were grown to exponential phase in rich media YM-1 containing 2% dextrose at 24 °C. To synchronize cells for early-hourglass analysis, bar1Δ (YEF2497) and bar1Δ CDC3-GFP (YEF7170) cells were grown to exponential phase in SC media lacking leucine (SC-Leu) but containing 2% dextrose at 24 °C and then treated with 50 ng ml −1 of α -factor [20] . The cells were incubated at 24 °C for 2 h until 99% of cells were synchronized in G1 as unbudded cells. Cells were washed three times with SC-Leu media without dextrose to remove pheromone and then resuspended in the same media with dextrose and incubated for another 45 min at 24 °C. For transition-structure and double-ring analysis, cdc15-2 (DL3034) and cdc15-2 CDC3-GFP (YEF7171) cells were grown in SC media with 2% dextrose and adenine sulfate (80 mg l −1 ), to the exponential phase, at 24 °C in a large volume (at least 300 ml). An equivalent volume of media pre-warmed to 37 °C was added to the culture and cells were put in an air incubator at 37 °C for 3 h. Cells for analysis of the transition structures were processed at this point. Synchrony at the transition stage in cdc15-2 myo1Δ and cdc15-2 shs1Δ mutants was achieved by the same method (YEF7406, YEF7453, YEF7486 and YEF7487). For double-ring analysis, cells were additionally incubated in a 24 °C water bath for 40 min. Synchrony for early hourglass, double ring and transition stages was assessed in CDC3-GFP strains after spheroplast processing (see below) without the addition of cell wall-digesting enzyme (zymolyase) so that the stage could be assessed by cell morphology and septin structure. This additionally allowed us to control for any progression through the cell cycle during the spheroplasting protocol. Spheroplasting Cells were spun at 23 °C (4,300 g for 5 min) and resuspended in 3.5 ml TE buffer (40 mM Tris, 40 mM EDTA, pH 8.0) and 17.5 μl β-mercaptoethanol per gram of cells. Cells were incubated at 30 °C for 15 min, then spun and washed once with spheroplast buffer (10 mM PIPES, 1 M sorbitol, pH 6.5). Cells were then spun and resuspended in 4 ml of spheroplast buffer per gram of cells. Fifty units of zymolyase 100T (Amsbio, Oxfordshire, UK) was added and the cells were incubated at 30 °C for 1 h. Spheroplasts were then spun at 4 °C and washed with chilled spheroplast buffer three times and finally resuspended at a concentration of 1–2 optical density at a wavelength of 600 nm (OD 600 ) per ml. Unroofing spheroplasts This method is adapted from Rodal et al. [19] Coverslips were coated with high-molecular-weight poly-lysine (Sigma Aldrich, St Louis, MO) by spotting on 10 μl of 1 mg ml −1 poly-lysine in water and incubating at 23 °C for 20 min. For correlative light/EM, coverslips that were marked with a gold-finder grid were used instead. The excess was aspirated off and the coverslip was spotted with sterile H 2 O. After aspirating off the water, the coverslip was allowed to dry for 30 min and was used within an hour. Coated coverslips were placed into 12-well plates and submerged in spheroplast suspension. The plate was spun at 3,000 r.p.m. for 5 min at 4 °C. The following solutions were prepared in four petri dishes: 1, spheroplast buffer; 2, KHMgE buffer (70 mM KCl, 20 mM HEPES, 5 mM MgCl 2 , 3 mM EGTA, pH 7.5); 3, KHMgE buffer; 4, KHMgE buffer. A spheroplast-coated coverslip was gently and quickly dipped into dishes 1 and 2, then placed into 3. This was repeated with another coverslip that was inverted onto the first coverslip in dish 3 such that the spheroplasts were sandwiched in between. Light force was applied to the two coverslips for 5 s with forceps, with care to avoid sliding between the two coverslips. The coverslips were gently separated again with care to avoid slippage and quickly dipped into dish 4 before being placed in fixative (KHMgE+2% EM grade glutaraldehyde) in a 12-well plate. Fixed, unroofed spheroplasts were stored up to a month before immunofluorescence or EM processing. Electron microscopy Sample processing for platinum-replica EM was performed as previously described [18] . In brief, glutaraldehyde-fixed, unroofed spheroplasts were further sequentially treated with tannic acid and uranyl acetate before ethanol dehydration and critical point drying. Dried samples were then rotary-shadowed at 45° angle with ~2 nm of platinum and at 90° angle with 3.5–5 nm of carbon. Coated samples were mounted on EM grids for analysis. EM samples were analysed using a JEM 1011 transmission electron microscope (JEOL USA, Peabody, MA) operated at 100 kV. Images were captured with an ORIUS 832.10W charge-coupled device (CCD) camera (Gatan, Warrendale, PA) and presented in inverted contrast. An Unsharp filter was used to sharpen EM images in the figures. Colour labelling of structures of interest was performed using the Hue/Saturation tool in Adobe Photoshop to avoid obscuring structural details. For correlative light and EM, immunofluorescence was performed on glutaraldehyde-fixed cortices prepared on gold-finder grid marked coverslips before EM processing. Antibody to Cdc11 (y-415, Santa Cruz Biotechnology, Dallas, TX) and Alexa Fluor 488 anti-rabbit IgG (A-21441, Life Technologies, Carlsbad, CA) were used at 1:100 and 1:500, respectively, diluted in PBS containing 1% BSA. Primary and secondary antibody incubations were both for 1.5 h. Immunofluorescence imaging was performed with an Eclipse Ti-U microscope (Nikon, Tokyo, Japan) equipped with a Nikon Apo TIRF 100 × numerical aperture (NA) 1.49 objective (Nikon). The images were acquired using Image-Pro Plus, version 7.0 (Media Cybernetics, Bethesda, MD), with an electron-multiplying CCD (EMCCD) camera (QuantEM 512SC, Photometrics, Tucson, AZ). The positions of intact rings were recorded with respect to fiducial markers so that they could be found again during EM imaging. Quantification of EM micrographs Filament lengths were measured by manual tracing using the segmented line tool in ImageJ. The radii of intact septin rings were determined by tracing around the ring with the segmented line tool and measuring the perimeter of the region. The radius was calculated from this rough circumference using the equation 2 πr . The thickness of septin single and double filaments was determined by a 5-pixel line scan orthogonal to the filament(s) and using the Plot Profile function in ImageJ to quantify the gray values along the line. Peaks in the graph corresponded to filaments and the approximate midpoint of each peak along the y axis (that is, the gray value) was used to determine the diameter of the filament. The diameter of the rough myosin filaments was determined by approximately tracing around a straight segment of filament using the polygon tool and adjusting the threshold until the entire filament was filled in. The thresholded area was measured within the traced region and divided by the length of the segment to give the average diameter of the filament. Live-cell imaging with FRAP Yeast strain YEF6021 ( CDC3-GFP NUP57-mCherry ) was grown to exponential phase in SC-Leu media containing 2% dextrose at 23 °C. For imaging, 1 ml of the culture was briefly centrifuged in an Eppendorf tube (~30 s,~5,000 g ). Cell pellet was resuspended in ~50 μl supernatant. Approximately 3 μl of the cell suspension was taken and spotted on a 2% agarose slab containing SC media+2% dextrose on a glass slide. A coverslip was gently pushed on top of the slab and sealed with nail polish. The slide was then used for live-cell imaging. For FRAP analysis of septin bars in shmooing cells, yeast strain YEF7170 ( bar1Δ CDC3-GFP ) was grown in SC-Leu media containing 2% dextrose+50 ng ml −1 α -factor for 3 h at 23 °C to induce shmoo formation. Cells were then concentrated by centrifugation as described above. Approximately 3 μl of the cell suspension was taken and spotted on a 2% agarose slab containing SC media+2% dextrose on a glass slide and then processed as above for live-cell imaging. Acquisition was performed at 23 °C on a spinning-disk confocal microscope system consisting of the microscope IX71 (Olympus), scanhead CSU10 (Yokogawa Corporation of America) and × 100 objective (1.4 NA, Plan S-Apochromat oil immersion; Olympus) using an electron multiplying charge-coupled camera (C9100-13; ImagEM, Hamamatsu Photonics). Lasers for excitation of green fluorescent protein (GFP; 488 nm) or mCherry/red fluorescent protein (RFP; 561 nm) were housed in a Spectral Applied Research launch. A computer-controlled ablation system (MicroPoint, Photonic Instruments) equipped with a nitrogen-pumped dye laser (435 nm) was used for FRAP. MetaMorph 7.7 software (Molecular Devices) controlled microscope and equipment, and was used for image acquisition. Images were taken at 1-min intervals, with a z stack consisting of 12 or 13 × 0.4-μm steps. Exposure time was set to 125 ms (GFP) or 150 ms (RFP), EM Gain to 150 (GFP) or 175 (RFP), and the Digitizer to 11 MHz. FRAP analysis Post-acquisition image analysis was performed in ImageJ (National Institutes of Health). An average projection for quantification or maximum projection for presentation was made. When too much cell movement occurred over the time of acquisition, stack registration was performed (rigid-body method) in ImageJ, using the plugin StackReg [37] . For quantification, a polygon fitting the region of interest (ROI; bleached or unbleached area) was drawn and the integrated density was calculated using ImageJ. In GraphPad Prism 5, the integrated density, relative to the starting point (before bleach), was calculated and plotted. Live-cell imaging with photoactivation and photoconversion For live-cell imaging with photoactivation or photoconversion, cells were cultured in SC-dropout (a specific amino acid or uracil was omitted) media to exponential phase at 23 °C. Cells were then embedded in a layer of medium solidified with 1.2% low-melting-temperature agarose (Lonza) in a poly-lysine-coated glass bottom dish (MatTek). Image acquisitions were performed on a microscope (Olympus, IX81) with a spinning-disk confocal scan head (Yokogawa, CSU-X1) and a × 100 objective lens (Olympus, 1.4 NA) using an EMCCD camera (Andor, iXon3). Image acquisition was controlled by MetaMorph (Molecular Devices). Two diode lasers (488 nm for GFP and 561 nm for RFP) were used for excitation illumination. Excitation laser intensities were set at 15% of the maximal output. For photoactivation and photoconversion, 405-nm laser was used at the minimum output intensity. The 405-nm laser was controlled via a plugin (iLas [2] , Roper Scientific) installed in MetaMorph. For photoactivation, 10 × 10-pixel regions set in the vicinity of the target cells were illuminated by the 405-nm laser with the settings of 100 repetitions × 3 times and thickness 5. For photoconversion, 2 × 2-pixel regions set in the vicinity of the target cells were illuminated by the 405-nm laser with the settings of 100 repetitions × 3 times and thickness 5. An on-chip EM gain setting of 200 was used for the EMCCD camera. Exposure time was set in a range from 150 to 200 ms per acquisition. Z -stacks were set as 11 × 0.6 μm to 11 × 0.7 μm. Acquisition intervals were set in a range from 1.5 to 2 min. Live-cell imaging with 3D-SIM For live-cell imaging with 3D-SIM, cells were cultured in SC-dropout media to exponential phase at 23 °C. Cells were then embedded in a layer of medium solidified with 1.2% low-melting-temperature agarose (Lonza) in a poly-lysine-coated glass bottom dish (MatTek). Image acquisitions were performed on a 3D-SIM super-resolution imaging system (DeltaVision OMX, Applied Precision) with a × 60 objective lens (Olympus, Plan-Apo, 1.42 NA). Image acquisition was controlled by softWoRx (Applied Precision). A 488-nm laser for GFP was used for excitation illumination. Excitation laser intensities were set at 10% of the maximal output. Camera gain was set as 1. Exposure time was set as 30 ms per acquisition. Z -stacks were set as 25 × 0.125 μm. Acquisition intervals were set at 3 min. Image processing and quantitative analysis of the photoactivation experiment Image processing and analysis were performed using Fiji [38] . For quantification of fluorescence intensities, image sequences generated by average projection were used. For quantification of fluorescence-signal-intensity kinetics after photoactivation, three ROIs with rectangular shape were set at photoactivated and un-photoactivated areas, and an area covering both. The integrated density was measured in each ROI. After subtraction of background signal and normalization by the value after septin hourglass splitting, the kinetics of the integrated density in each ROI was plot in a graph using Microsoft Excel. How to cite this article: Ong, K. et al. Architecture and dynamic remodelling of the septin cytoskeleton during the cell cycle. Nat. Commun. 5:5698 doi: 10.1038/ncomms6698 (2014).